m6A modification of a 3′ UTR site reducesRME1mRNA levels to promote meiosis Despite the vast number of modification sites mapped within mRNAs, known examples of consequential mRNA modifications remain rare. Here, we provide multiple lines of evidence to show that Ime4p, an N 6-methyladenosine (m 6 A) methyltransferase required for meiosis in yeast, acts by methylating a site in the 3′ UTR of the mRNA encoding Rme1p, a transcriptional repressor of meiosis. Consistent with this mechanism, genetic analyses reveal that IME4 functions upstream of RME1 . Transcriptome-wide, RME1 is the primary message that displays both increased methylation and reduced expression in an Ime4p-dependent manner. In yeast strains for which IME4 is dispensable for meiosis, a natural polymorphism in the RME1 promoter reduces RME1 transcription, obviating the requirement for methylation. Mutation of a single m 6 A site in the RME1 3′ UTR increases Rme1p repressor production and reduces meiotic efficiency. These results reveal the molecular and physiological consequences of a modification in the 3′ UTR of an mRNA. N 6 -methyladenosine (m 6 A), one of the hundreds of posttranscriptional RNA modifications known to occur in RNA [1] , is the most common internal modification in eukaryotic mRNA [2] , [3] . The mRNA methyltransferase is a protein complex in which one of its members, encoded by the IME4 gene in yeast (Initiator of MEiosis 4), harbors the catalytic activity [4] . In many yeast strains, IME4 is required for progression through meiosis [5] , [6] , and the recognition that it encodes an mRNA methyltransferase has provided the initial evidence that internal mRNA modifications have physiological consequences [4] . Ime4p is conserved among eukaryotes, with characterized homologs in mammals (METTL3) [7] , Drosophila (dIME4) [8] , and Arabidopsis (MTA) [9] . Other noncatalytic members of the yeast methyltransferase complex include Slz1p and Mum2p [10] , [11] . MUM2 also has homologs in mammals (WTAP) [12] , [13] , Drosophila (Fl(2)d) [14] , and Arabidopsis (FIP37) [9] , [15] . The m 6 A mark is found in a conserved consensus motif within mRNAs [16] , [17] and thought to be deposited co-transcriptionally based on its presence in chromatin-associated pre-mRNA exons [18] , co-localization of dIme4 and PolII on Drosophila chromosomes [19] , and increased m 6 A levels in transcripts with reduced transcription rates [20] . m 6 A is most often found in proximity to stop codons, in either the coding sequence or the 3′ untranslated region (UTR) [21] , [22] , [23] , and has been broadly linked to diverse aspects of mRNA metabolism and function, including altered splicing [19] , [24] , [25] , [26] , decreased mRNA stability [27] , [28] , [29] , and altered translational efficiency [20] , [28] , [30] , [31] , [32] . Some of the consequences of m 6 A mRNA methylation rely on “reader” proteins, which have a YTH domain that interacts specifically with m 6 A [33] , [34] , [35] , [36] , [37] . YTHDF1 and YTHDF3 bind to a subset of m 6 A mRNAs and enhance their translation, and in the case of YTHDF1 this increased translation efficiency results from its interaction with members of the eIF3 complex [26] , [38] . YTHDF2 is implicated in mRNA degradation, as its knockdown results in increased mRNA half-life of m 6 A mRNAs [29] . Deletion of YTHDF2 in mice results in female infertility [39] . Similarly, YTHDC2 deletion in mice results in infertility due to meiotic arrest during gametogenesis [40] . In Drosophila, dIME4 is expressed in gonads and required for gametogenesis [8] . When considered together with the ime4 - Δ phenotype in yeast, these results suggest that m 6 A has an evolutionarily conserved role in meiosis. Meiosis in S. cerevisiae is part of the sporulation-differentiation program, in which four haploid spores are formed from one diploid cell [41] . The decision to enter meiosis is controlled through multiple pathways that integrate nutritional and ploidy signals. Diploid cells enter meiosis when starved for nitrogen in the presence of a non-fermentable carbon source. The master regulator of meiosis in yeast is a transcriptional activator called Initiator of meiosis 1 (Ime1p). IME1 has one of the longest promoters in the yeast genome, which harbors binding sites for proteins that transmit the nutritional status signals [42] and two binding sites for Rme1p (Regulator of meiosis 1), a DNA-binding protein that prevents meiosis in haploids by repressing IME1 transcription [43] , [44] , [45] , [46] . In diploids, RME1 is itself repressed by the product of the mating-type alleles, the a1/α2 complex [44] . However, genetic and mutational analyses suggest that there are additional unidentified mechanisms of RME1 repression [44] . IME4 , which encodes the mRNA m 6 A methyltransferase in yeast, is known to be required for IME1 expression, but how this positive regulation is achieved has been unclear [6] . Furthermore, it is unclear why IME4 is necessary for meiosis in some yeast strains [6] but dispensable in others [10] . The regulatory impact of m 6 A modifications within mRNAs, inferred from phenotypic and molecular analyses of mutations that disrupt m 6 A writers or readers in yeast, plants, flies, and mammals, is now broadly appreciated [47] , [48] , [49] . Less progress has been made in distinguishing the consequential m 6 A sites out of the entire m 6 A methylome. Thus far, one functional m 6 A modification has been reported in an intron of the mammalian S-adenosylmethionine (SAM) synthase mRNA, which regulates its splicing [25] , [50] . Two functional m 6 A sites were reported in the 5′ UTRs of mammalian HSP70 and ATF4 , where they regulate cap-independent translation and alternative translation, respectively [51] , [52] . However, the vast majority of mapped m 6 A sites are near the stop codon and at the 3′ UTR [21] , [22] , for which there are no known physiologically relevant examples validated by mutational analysis. In this study, we identify a consequential m 6 A site within the RME1 3′ UTR that reduces RME1 mRNA levels to enable meiotic progression. Thus IME4 lies upstream of RME1 in the meiotic entry pathway, which explains the decades-old observation that IME4 is required for IME1 expression. These results reveal the molecular consequences of a modification in the 3′ UTR of an mRNA and explain the strain-dependent requirement for methylation of mRNA. A promoter polymorphism reduces RME1 expression Polymorphisms in several genes account for most of the difference in meiotic efficiency between two interbreeding strains of Saccharomyces cerevisiae : SK1 (high efficiency) and S288C (low efficiency) [53] , [54] . An S288C strain that has three alleles replaced with SK1 alleles—named SK288C—approaches SK1 in its elevated meiotic efficiency [54] , [55] . The SK1 allele with the largest contribution to meiotic efficiency is RME1-SK1 , which differs in sequence from that of rme1-S288C by three nucleotides [54] . One of these polymorphisms, insertion of an A (ins-308A, Fig. 1a ) located in the upstream non-coding region of RME1 , is solely responsible for efficient meiotic sporulation [54] . We named this allele RME1-SK1A and the allele in S288C rme1-S288C . Reverse transcription followed by quantitative PCR (RT-qPCR) showed that RME1-SK1A expression is reduced nearly four-fold compared with the rme1-S288C allele (Fig. 1b ), which is the allele present in most sequenced laboratory strains (Supplementary Fig. 1a ). Because Rme1p is a DNA-binding protein that directly represses the meiotic transcriptional program, this reduced transcription of RME1 explains the increase in meiotic efficiency in SK1. Our following studies on IME4 function utilize the SK288C strain, containing the highly expressed rme1-S288C , the poorly expressed RME1-SK1 allele, or a deletion of the entire RME1 -coding region ( RME1-Δ ). Fig. 1 RME1 alleles in this study. IME4 downregulates Rme1p through its m 6 A activity. a The three RME1 alleles are in the SK288C strain background. RME1-SK1A has a single A insertion 308 nucleotide upstream of the open reading frame (ORF) relative to rme1-S288C . b Quantitative reverse transcription PCR (RT-qPCR) quantification of RME1-SK1A and rme1-S288C expression during meiosis. Means and individual values from three biological replicates. Source data are provided in a Source Data file. c m 6 A immunoprecipitation (IP) followed by RT-qPCR using RME1 5′ untranslated region (UTR) primers or primers that span the end of the ORF and the 3′ UTR on mRNA isolated from IME4 and ime4-cat homozygous cells, both in rme1-S288C homozygous cells. Transcript levels were first normalized to PGK1 as an internal control, and then the fold enrichment of IP/input was calculated. The residual enrichment of RME1 transcripts in ime4-cat / ime4-cat cells relative to IME4 / IME4 cells probably results from non-specific binding to the anti-m 6 A antibody [13] , [23] . ACT1 serves as a non-methylated control. Means, individual values, and s.d. from three biological replicates. * p = 0.022, ** p = 0.019, two-tailed t test. Source data are provided in a Source Data file. d Western blot using anti-FLAG antibody showing Rme1p expression from the rme1-S288C allele in strains homozygous for the indicated allelic backgrounds incubated in SPO media for 5 h. A non-specific (NS) band present in all lanes serves as a loading control. Source data are provided in a Source Data file Full size image IME4 represses Rme1p expression SK1 and S288C differ because IME4 is essential for meiosis in S288C but dispensable for meiosis in SK1 (Supplementary Fig. 1b [10] ). IME4 encodes a methyltransferase that directs the posttranscriptional conversion of A to m 6 A in mRNA [4] . To determine whether the differential IME4 dependence is due to a role for Ime4p and/or m 6 A in regulating RME1 expression, we generated a strain homozygous for a deletion of IME4 ( ime4-Δ / ime4-Δ ) and a strain homozygous for a catalytically inactive allele ( ime4-cat / ime4-cat ) [4] . The Ime4p and ime4p-cat proteins were expressed to the same levels during meiosis and vegetative growth (Supplementary Fig. 1c ). m 6 A immunoprecipitation (m 6 A IP) of mRNA purified from meiotic IME4 / IME4 and ime4-cat / ime4-cat cells captured less RME1 mRNA from ime4-cat / ime4-cat lysate, suggesting that RME1 transcripts carried the m 6 A modification (Fig. 1c ). Does methylation of RME1 mRNA affect the expression of Rme1p? We found that both ime4-Δ / ime4-Δ and ime4-cat / ime4-cat cells had increased Rme1p levels relative to IME4 / IME4 (Fig. 1d and Supplementary Fig. 1d ). IP confirmed the increase in Rme1p in these cells (Supplementary Fig. 1e ). Rme1p appeared to be posttranslationally modified in meiosis to produce higher-molecular-weight species (Supplementary Fig. 1d ). These higher-molecular-weight forms of Rme1p were dithiothreitol (DTT)-resistant, migrate too fast to be sodium dodecyl sulfate (SDS)-resistant homo-oligomers, and did not react with anti-ubiquitin antibodies (Supplementary Fig. 1e ). Thus Ime4p is required both for the methylation of RME1 mRNA and for reduced expression of Rme1p during meiosis. Ime4p reduces RME1 mRNA levels To reduce Rme1p levels, Ime4p catalytic activity might alter either mRNA levels or translational efficiency. To distinguish between these possibilities, we separated the actively translating pool of mRNA from total mRNA by sucrose-gradient polysome fractionation of IME4 / IME4 and ime4-cat / ime4-cat meiotic lysates. Compared to mitotic cells, meiotic cells had a marked reduction in polysomes (Fig. 2a ) [56] . Nonetheless, IME4 / IME4 and ime4-cat / ime4-cat cells exhibited comparable meiotic polysome profiles (Fig. 2b ), indicating that loss of m 6 A did not affect the ribosomal landscape. RNA-seq of the input and polysome fraction revealed that the total levels of RME1 mRNA were increased in ime4-cat / ime4-cat cells compared to IME4 / IME4 cells and that there was no further increase in polysome-associated RME1 mRNA (Fig. 2c ). Therefore, the increase in Rme1p can be explained by the increase in RME1 mRNA. Parallel analyses of other mRNAs showed that such an increase in mRNA was unusual and not observed for >98% of the other mRNAs (Fig. 2d ). Taken together, these data indicate that Ime4p catalytic activity specifically decreases Rme1p production by reducing transcript abundance rather than polysome association. Fig. 2 IME4 m 6 A activity reduces RME1 mRNA levels to enable meiotic initiation. a Polysome profiles (absorbance at 254 nm vs. distance from the top of the tube) of mitotic cells during logarithmic growth and 2 h into meiosis. The locations of the 40S, 60S, monosome, and polysome peaks are indicated. Source data are provided in a Source Data file. b Polysome profiles of meiotic IME4 / IME4 and ime4-cat / ime4-cat cells, both in rme1-S288C / rme-S288C . The inset is a magnification of the polysome area with the number of ribosomes in each peak. The highlighted area marks the pooled fractions used for RNA-seq of polysome-associated mRNA. Source data are provided in a Source Data file. c RNA-seq quantifications of RME1 transcript from input mRNA prior to gradient fractionation (total mRNA) and pooled polysome fractions (polysomal RNA) from IME4 / IME4 and ime4-cat / ime4-cat meiotic cells. Individual values, means, and s.d. from three biological replicates. Two-way analysis of variance p values are indicated. Source data are provided in a Source Data file. d Rank order plot of mRNA levels in total RNA from ime4-cat / ime4-cat and IME4 / IME4 meiotic cells. Means from three biological replicates. Source data are provided in a Source Data file. e Left: Quantitative reverse transcription PCR (RT-qPCR) quantification of IME1 expression in RME1-Δ / RME1-Δ during meiosis in IME4 / IME4 and ime4-Δ / ime4-Δ cells. Middle: RT-qPCR quantification of IME1 expression in rme1-S288C / rme1-S288C during meiosis in IME4 / IME4 and ime4-Δ / ime4-Δ cells. Right: RT-qPCR quantification of IME1 expression in rme1-S288C / rme1-S288C during meiosis in IME4 / IME4 and ime4-cat / ime4-cat cells. Means and individual values from three biological replicates. Source data are provided in a Source Data file. f As in e above but with measurements of IME2 expression. Means and individual values from three biological replicates. Source data are provided in a Source Data file Full size image RME1 repression enables the meiotic transcriptional program Rme1p blocks meiosis by preventing activation of the IME1 gene, which encodes the master transcriptional activator of meiosis [42] , [57] , [58] , [59] . IME1 is necessary for meiotic DNA replication [57] , [60] , even in the presence of the RME1-SK1A allele (Supplementary Fig. 1f ). To test whether reduced RME1 mRNA de-represses IME1 , the level of IME1 mRNA was determined by RT-qPCR in IME4 / IME4 , ime4-Δ / ime4-Δ , and ime4-cat / ime4-cat cells. As expected, in the RME1-Δ / RME1-Δ background, we observed no difference in IME1 mRNA levels between IME4 / IME4 and ime4-Δ / ime4-Δ cells after 5 h in SPO media (Fig. 2e ). By contrast, in the rme1-S288C / rme1-S288C background, IME1 levels were reduced more than three-fold in both ime4-Δ / ime4-Δ and ime4-cat / ime4-cat cells relative to IME4 / IME4 cells (Fig. 2e ). Analysis of the time courses showed that an initial burst of IME1 expression was induced equally in IME4 / IME4 , ime4-Δ / ime4-Δ , and ime4-cat / ime4-cat cells, but ime4-Δ / ime4-Δ and ime4-cat / ime4-cat cells failed to sustain elevated IME1 expression. This role of Ime4p in sustaining high-level IME1 expression by overcoming Rme1p repression coincided with the timing of its induced expression (Supplementary Fig. 1c ). We observed an increase in IME1 mRNA levels in early time points in IME4 / IME4 compared to ime4-Δ / ime4-Δ cells in the RME1-Δ / RME1-Δ background. This increase suggests that Ime4p has an additional role in IME1 regulation independent of RME1 (Fig. 2e ), although this role was not further investigated. Perhaps Ime4p is involved in transduction of the nutritional starvation signals required to induce IME1 [42] , [61] . One of the target genes induced by Ime1p is IME2 , which encodes a protein kinase required for the expression of many other meiotic genes [58] , [59] , [62] . IME2 expression in the different RME1 backgrounds paralleled that of IME1 , indicating that the effects of Ime4p regulation of RME1 propagate through IME1 induction to activate the downstream meiotic targets (Fig. 2f ). A conditional IME4 requirement for meiotic DNA replication The transcriptional program induced in meiosis initially consists of genes required to carry out meiotic DNA replication. As a functional readout of this process, we measured DNA content by flow cytometry in IME4 / IME4 , ime4-Δ / ime4-Δ , and ime4-cat / ime4-cat cells in the RME1-Δ , RME1-SK1A , and rme1-S288C homozygous backgrounds following 6 and 24 h in SPO media (Fig. 3a ). Deletion of IME4 led to delayed meiotic DNA replication in cells with no or low RME1 expression ( RME1-Δ and RME1-SK1A , respectively). However, in the presence of high RME1 expression ( rme1-S288C ), we detected no DNA replication in ime4-Δ / ime4-Δ cells, even after 24 h. Cell sorting followed by microscopy revealed that cells to the right of the 4 N peak at 24 h were asci (Supplementary Fig. 2a, b ). The DNA-replication defect observed in ime4-Δ / ime4-Δ cells was not quite as severe in ime4-cat / ime4-cat cells. Although DNA replication was substantially delayed in ime4-cat / ime4-cat cells in the rme1-S288C background, some cells ultimately were able to replicate their DNA. Thus the ime4-cat allele was incompletely penetrant, suggesting that Ime4p might perform both methyltransferase-dependent and -independent functions. Fig. 3 IME4 m 6 A is required for meiotic DNA replication, and a non-m 6 A function is required for meiotic divisions. a Flow cytometric analysis of DNA content in IME4 and ime4 mutants (rows) in three color-coded RME1 allele backgrounds over a meiotic time course (columns). A quantification of the 24-h time point is on the right of each row. Percentage of cells with 4 N includes both sporulated and non-sporulated cells. Means, individual values, and s.d. from two to five experiments. Source data are provided in a Source Data file. b Meiotic nuclear divisions in IME4 and ime4 mutants in three color-coded RME1 allele backgrounds as assayed by DAPI staining of nuclei after 24 h in SPO medium. The percentage of cells with two or more nuclei is indicated on the horizontal axis. Means, individual values, and s.d. from three experiments. At least 200 cells were counted per strain per experiment. Source data are provided in a Source Data file. c Sporulation after 48 h in SPO media in IME4 and ime4 mutants in three color-coded RME1 allele backgrounds as scored by light microscopy. Means, individual values, and s.d. from three experiments. At least 200 cells were counted per strain per experiment. Source data are provided in a Source Data file. d A model depicting the various points along the S. cerevisiae meiotic program in which different IME4 functions are needed in different RME1 backgrounds. “ RME1 on” denotes the highly expressed rme1-S288C allele, while “ RME1 off” denotes either the hypomorph RME1-SK1A or RME1-Δ . Arrows represent an ability to progress through the various landmarks that appear at the top, while vertical red lines indicate an inability to progress further. e A model for the functions of IME4 in meiosis: IME4 promotes meiotic DNA replication by repression of RME1 , which represses the master activator of meiosis, IME1 . IME1 is also activated by nutritional signals. IME4 has a second function downstream of IME1 in promoting meiotic divisions (dashed line) Full size image If IME4 and RME1 were in the same pathway, then the DNA-replication phenotypes of the single- and double-deletion strains would indicate their order in the pathway and whether they activate or inhibit each other (Supplementary Table 3 lists the predicted phenotypes for each of the eight possible models). For this analysis, a double-deletion strain of RME1 and IME4 was constructed, and meiotic DNA synthesis was measured and compared with that of the wild-type RME1 and IME4 strain and the respective single-deletion strains (Fig. 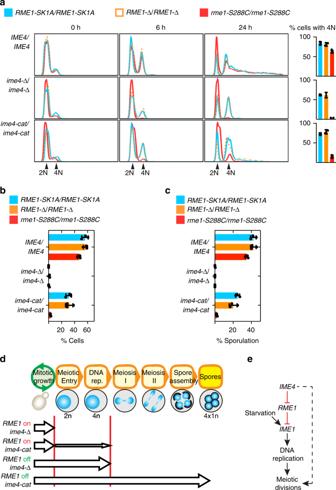Fig. 3 IME4m6A is required for meiotic DNA replication, and a non-m6A function is required for meiotic divisions.aFlow cytometric analysis of DNA content inIME4andime4mutants (rows) in three color-codedRME1allele backgrounds over a meiotic time course (columns). A quantification of the 24-h time point is on the right of each row. Percentage of cells with 4Nincludes both sporulated and non-sporulated cells. Means, individual values, and s.d. from two to five experiments. Source data are provided in a Source Data file.bMeiotic nuclear divisions inIME4andime4mutants in three color-codedRME1allele backgrounds as assayed by DAPI staining of nuclei after 24 h in SPO medium. The percentage of cells with two or more nuclei is indicated on the horizontal axis. Means, individual values, and s.d. from three experiments. At least 200 cells were counted per strain per experiment. Source data are provided in a Source Data file.cSporulation after 48 h in SPO media inIME4andime4mutants in three color-codedRME1allele backgrounds as scored by light microscopy. Means, individual values, and s.d. from three experiments. At least 200 cells were counted per strain per experiment. Source data are provided in a Source Data file.dA model depicting the various points along theS. cerevisiaemeiotic program in which differentIME4functions are needed in differentRME1backgrounds. “RME1on” denotes the highly expressedrme1-S288Callele, while “RME1off” denotes either the hypomorphRME1-SK1AorRME1-Δ. Arrows represent an ability to progress through the various landmarks that appear at the top, while vertical red lines indicate an inability to progress further.eA model for the functions ofIME4in meiosis:IME4promotes meiotic DNA replication by repression ofRME1, which represses the master activator of meiosis,IME1.IME1is also activated by nutritional signals.IME4has a second function downstream ofIME1in promoting meiotic divisions (dashed line) 3a ). Only the double-repression model, in which IME4 acts upstream to repress RME1 , which in turn represses DNA replication, explained all the single- and double-deletion experimental data (Supplementary Table 3 ). IME4 is known to be required for the expression of IME1 [6] . Our results show that this positive genetic relationship is achieved via negative regulation of RME1 (Fig. 3e ). RME1 dosage tightly controls meiotic DNA replication Our observation that the ~3–4-fold reduction in RME1 expression caused by the RME1-SK1A allele (as compared to rme1-S288C , Fig. 1b ) had a dramatic effect on meiotic efficiency suggests that the downstream events in meiosis are sensitive to RME1 dosage. To examine the effects of RME1 transcript levels on meiotic progression, we analyzed DNA synthesis in various strains. Heterozygotes containing half the amount of rme1-S288C ( rme1-S288C / RME1-Δ ) replicated their DNA earlier than rme1-S288C homozygotes (Supplementary Fig. 3a ). Furthermore, in the absence of IME4 ( ime4-Δ / ime4-Δ ), rme1-S288C / RME1-Δ cells replicated their DNA, whereas rme1-S288C / rme1-S288C did not. These data demonstrate that a two-fold reduction in RME1 levels is sufficient to bypass the meiotic defects of a deletion of IME4 . Moreover, heterozygotes containing one copy of the poorly expressed RME1-SK1A allele and one copy of the highly expressed rme1-S288C allele ( ime4-Δ / ime4-Δ RME1-SK1A / rme1-S288C ) proceeded through DNA replication, whereas ime4-Δ / ime4-Δ rme1-S288C / rme1-S288C homozygotes did not (Supplementary Fig. 3b ). Consistent with these results, in strains homozygous for the ime4-cat allele, rme1-S288C / RME1-Δ and RME1-SK1A / rme1-S288C heterozygotes replicated their DNA earlier than rme1-S288C homozygotes. A methyltransferase activity-independent Ime4p function We monitored segregation of DNA into distinct nuclei by microscopy and found that, in ime4-Δ / ime4-Δ cells, no meiotic divisions occurred in any RME1 allelic background (Fig. 3b and Supplementary Fig. 3c ). This indicates that IME4 is required downstream of DNA replication for the onset of Meiosis I. However, Ime4p catalytic activity was not required for DNA segregation: meiotic divisions occurred efficiently in ime4-cat / ime4-cat cells, provided they were able to replicate their DNA ( RME1-Δ or RME1-SK1A backgrounds). Analysis of sporulation efficiency showed that it precisely mirrored DNA segregation in the ime4 mutants in the various RME1 backgrounds (Fig. 3c and Supplementary Fig. 3c ). We conclude that, in the presence of an active RME1 allele, ime4-Δ / ime4-Δ cells do not replicate their DNA, whereas ime4-cat / ime4-cat cells are severely defective in DNA replication and those that do replicate their DNA arrest following DNA replication (Fig. 3d ). In the absence of an active RME1 allele, ime4-Δ / ime4-Δ cells arrest following DNA replication, whereas ime4-cat / ime4-cat cells are able to complete meiosis and sporulate. Together these data reveal that Ime4p functions twice during meiosis: once as an m 6 A methyltransferase that promotes DNA replication, and again before Meiosis I in a catalysis-independent manner to promote DNA segregation (Fig. 3e ). RME1 mRNA is an m 6 A target To identify Ime4p methylation targets critical for progression of the meiotic program, we performed m 6 A IP followed by RNA-seq (m 6 A-seq) [21] , [22] on RNA from the 5-h meiotic time point of rme1-S288C / rme1-S288C cells, in which Ime4p catalytic activity is necessary for meiosis. This m 6 A-seq experiment contrasts with previous analyses performed in the SK1 background, where Ime4p m 6 A activity is dispensable for meiosis [23] . We identified 118 sites on 117 transcripts enriched in IME4 / IME4 cells relative to ime4-cat / ime4-cat cells (Supplementary Data 1 , see “Methods”). Using these data, we reconstructed the known m 6 A methylation consensus motif and reproduced the observation that m 6 A sites are enriched near the 3′ ends of mRNAs (Supplementary Fig. 4a–c ) [21] , [22] , [23] . Of the 117 methylated mRNAs we identified, 51 were also identified in the previous m 6 A-seq dataset from the meiotic-efficient SK1 (Supplementary Fig. 4d , p < 0.0001, Fisher’s Exact Test [23] ). Analysis leveraging our biological replicates revealed 34 high-confidence m 6 A sites on 34 different mRNAs in IME4 / IME4 cells compared with ime4-cat / ime4-cat cells (log 2 fold change >0.8, p < 0.01, two-tailed t test) (Fig. 4a and Supplementary Data 1 ). The set of high-confidence m 6 A targets included RME1 . Fig. 4 RME1 mRNA harbors an m 6 A site at its 3′ untranslated region (UTR). a m 6 A-seq data from meiotic IME4 homozygotes and ime4-cat homozygotes. Data from three biological replicates are presented as immunoprecipitation (IP) to input ratio in IME4 , divided by the same ratio in ime4-cat . m 6 A sites enriched >1.75-fold in IME4 relative to ime4-cat cells that have a p value of <0.01 in a two-tailed t test are highlighted in orange. b RNA-seq data from meiotic IME4 homozygotes and ime4-cat homozygotes cells. Data from three biological replicates are presented as normalized counts in ime4-cat , divided by normalized counts in IME4 . mRNAs increased >1.75-fold in ime4-cat / ime4-cat relative to IME4 / IME4 cells ( p value <0.01, two-tailed t test) are highlighted in purple. mRNAs decreased >1.75-fold in ime4-cat / ime4-cat relative to IME4 / IME4 cells ( p value < 0.01, two-tailed t test) are highlighted in blue. c Venn diagram showing the overlap between the m 6 A-seq data and the RNA-seq data. d RME1 transcript with its 5′ and 3′ UTRs. IGV genome browser views of reads enriched following IP with anti-m 6 A antibodies in IME4 / IME4 and ime4-cat / ime4-cat cells are shown for the entire transcript (top, autoscale read counts on the left of each track), and in a 100-bp window of the 3′ UTR (bottom, reads in this window were normalized to input controls). Fold enrichment of IP/input for reads in the window are shown on the left with means and s.d. from three biological replicates. * p = 0.0006, two-tailed t test. Source data are provided in a Source Data file. e PCR amplification of cDNA prepared from MazF-digested meiotic mRNA from IME4 / IME4 and ime4-cat / ime4-cat cells. Three biological replicates. P1 and P2 primer locations relative to the probed methylation site are indicated. The MazF ACA site within the methylation site is highlighted in yellow, and the probed nucleotide is marked with an asterisk. Primers P3 and P4, which do not flank an ACA site, were used as control. Source data are provided in a Source Data file Full size image In a separate experiment using rme1-S288C / rme1-S288C cells at the 5-h meiotic time point, we also measured the global mRNA levels of IME4 / IME4 and ime4-cat / ime4-cat cells. Analysis of these RNA-seq data revealed 97 mRNAs with significantly elevated levels (log 2 fold change >0.8, p < 0.01, two-tailed t test) in ime4-cat / ime4-cat cells relative to IME4 / IME4 cells (Fig. 4b and Supplementary Data 2 ). These 97 transcripts were enriched for ribosome- and amino acid synthesis-related gene ontologies (GOs; Supplementary Fig. 5a ). Parallel analysis of the 156 mRNAs elevated in IME4 / IME4 cells relative to ime4-cat / ime4-cat cells revealed enrichment for meiosis-related categories including synapsis, recombination, homologous chromosome segregation, and sister-chromatid segregation (Supplementary Fig. 5b ). Remarkably, the intersection of the set of 97 messages elevated in the absence of Ime4p methyltransferase activity with the set of 34 high-confidence m 6 A targets contained one gene: RME1 (Fig. 4c ). Mutation of RME1 3′ UTR m 6 A site increases its mRNA levels A parsimonious explanation for our results so far is that Ime4p directly methylates RME1 mRNA at a specific site, and the m 6 A mark reduces RME1 mRNA stability. Analysis of the m 6 A-seq data indeed revealed a single significant peak in the RME1 message located in the 3′ UTR that was enriched three-fold in IME4 / IME4 cells relative to ime4-cat / ime4-cat cells (Fig. 4d ). This peak is centered on a putative m 6 A site 129 nt downstream of the stop codon (+129A), which matched the consensus m 6 A motif (ANRG-m 6 A-CNNU). In order to probe the methylation status of +129A, we used MazF, a methylation-sensitive RNA restriction enzyme [63] , in a recently described PCR-based assay [64] . MazF cleaves RNA at ACA sites but not at m 6 ACA sites. The ACA sequence is part of the GG ACA sequence flanking +129A (Fig. 4e ). We digested purified mRNA from IME4 / IME4 and ime4-cat / ime4-cat cells with MazF and then reverse transcribed with random hexamers. PCR amplification of the resulting cDNA using primers that flank +129A in the RME1 3′ UTR yielded a product in cDNA prepared from IME4 / IME4 but not from ime4-cat / ime4-cat (Fig. 4e ). Thus +129A in the RME1 3′ UTR is protected from cleavage by MazF in mRNA derived from cells with a functional methyltransferase. This result confirms that the RME1 3′ UTR is methylated at the +129A position in IME4 / IME4 cells but not in ime4-cat / ime4-cat cells. To determine whether methylation of this +129A was important for RME1 regulation, we mutated the A to a T in the RME1 genomic locus (Fig. 5a , rme1-10 ). RNA-seq of rme1-10 / rme1-10 cells showed a significant increase in total RME1 mRNA levels and polysomal mRNA levels relative to rme1-S288C / rme1-S288C (Fig. 5b ). Transcriptome-wide analysis of mRNAs in rme1-10 / rme1-10 and rme1-S288C / rme1-S288C meiotic cells revealed that RME1 was among the most differentially expressed genes (1.46-fold induction, p = 0.003, two-tailed t test, Fig. 5c ). Comparison of rme1-10 / rme1-10 and ime4-cat / ime4-cat cells revealed a significant correlation in mRNA expression levels across the transcriptome (Supplementary Fig. 5c ). When compared to wild-type cells ( IME4 / IME4 rme1-S288C / rme1-S288C ), these mutants shared an increase in mRNAs belonging to ribosome- and amino acid synthesis-related ontologies and a decrease in mRNAs belonging to nucleosome- and replication fork-related ontologies (Supplementary Fig. 5d, e )—hallmarks of proliferating cells. Fig. 5 RME1 methylation mutants are defective in meiotic DNA replication. a rme1-S288C and rme1-10 have the same promoter and coding sequence, but they differ in their 3′ untranslated region: rme1-10 has a single A to T substitution of the +129 methylated A (marked with an m over it) in the methylation consensus motif (yellow). b RNA-seq quantifications of RME1 mRNA. RME1 mRNA from input RNA prior to gradient fractionation (total mRNA) and polysome-associated RNA (polysomal RNA) from IME4 / IME4 rme1-S288C / rme1-S288C and IME4 / IME4 rme1-10 / rme1-10 cells incubated in SPO media for 5 h. Individual values, means, and s.d. from three biological replicates. Two-way analysis of variance p values are indicated. Because this experiment was performed together with the one shown in Fig. 2c , the results for RME1 mRNA in the IME4 background in Fig. 2c are re-plotted in this panel for the rme1-S288C background. Source data are provided in a Source Data file. c RNA-seq data from rme1-S288C homozygotes and rme1-10 homozygotes incubated for 5 h in SPO media. Data from three biological replicates are presented as normalized counts in rme1-10 , divided by normalized counts in rme1-S288C . d Flow cytometric analysis of DNA content over a meiotic time course in IME4 / IME4 rme1-10 / rme1-10 compared to IME4 / IME4 rme1-S288C / rme1-S288C and ime4-cat / ime4-cat rme1-S288C / rme1-S288C . Cells were incubated for 24 h at 30 °C or 37 °C, as indicated. Means, individual values, and s.d. from three biological replicates. * p = 0.011, ** p = 0.034, two-tailed t test. Source data are provided in a Source Data file Full size image RME1 3′ UTR m 6 A regulates meiotic DNA replication As expected from increased Rme1p production, IME4 / IME4 rme1-10 / rme1-10 cells were defective in DNA replication compared to IME4 / IME4 rme1-S288C / rme1-S288C cells (Fig. 5d ). The DNA-replication defect was less severe than that of ime4-cat / ime4-cat S288C / rme1-S288C cells, suggesting that the m 6 A activity of Ime4p also acts on other targets (or other sites on RME1 ) to promote meiotic DNA synthesis. Nonetheless, the single-nucleotide substitution in the m 6 A site of rme1-10 was sufficient to reduce meiotic DNA replication by 24%, accounting for nearly one third of the replication defect due to complete loss of m 6 A in ime4-cat / ime4-cat cells. The effect of rme1-10 was even greater at 37 °C, a restrictive temperature that decreases meiotic efficiency: me1-10 / rme1-10 cells had a 38% reduction in DNA replication compared to IME4 / IME4 cells, accounting for half of the replication defect in ime4-cat / ime4-cat cells. Thus this single m 6 A site within RME1 is required to dampen Rme1p production and enable efficient meiosis. The presence of the RME1-S288C allele in most laboratory strains including S288C, Sigma127b, W303, and RM11 (Supplementary Fig. 1a ) suggests that these strains have been selected for a strict mitosis–meiosis dichotomy. The highly sporulating SK1 is an outlier among laboratory strains as it carries the hypomorphic RME1-SK1A allele, which has a promoter mutation that reduces transcription of the RME1 repressor. Our data show that the requirement for IME4 and its catalytic methyltransferase function for meiosis is dependent upon the particular allele of RME1 carried by a strain. The SK288C strain is an excellent host for this analysis because it can be assessed for meiotic proficiency either with the fully functional rme1-S288C allele or with the hypomorphic RME1-SK1 allele. In a strain carrying the rme1-S288C allele, Ime4p and its catalytic methyltransferase function are required for efficient meiosis: meiotic DNA replication is abolished in ime4-Δ / ime4-Δ cells and severely reduced in ime4-cat / ime4-cat cells (Fig. 3a ). By contrast, meiotic DNA replication proceeds effectively in a strain carrying the RME1-SK1A allele without IME4 function ( ime4-Δ / ime4-Δ ), albeit at a slightly reduced rate. These results show that meiotic mRNA methylation is required only when RME1 is highly expressed; IME4 function is necessary to overcome repression of the meiotic program enforced by high levels of RME1 mRNA. Moreover, a small difference in RME1 transcription (two-fold) has a dramatic effect on meiotic DNA synthesis, implying that meiotic progression is very sensitive to the levels of RME1 (Supplementary Fig. 3a, b ). Ime4p m 6 A methyltransferase activity is needed to reduce expression of RME1 mRNA (Fig. 2c ). This downregulation is important because expression of RME1 mRNA continues throughout meiosis (Fig. 1b ) [65] . Given the posttranscriptional nature of the m 6 A modification, the lower mRNA expression level is presumably mediated by the destabilization of modified RME1 mRNA. Rme1p represses IME1 , the transcriptional activator of meiosis; consequently, downregulation of RME1 enables meiotic entry by relieving repression of IME1 and permitting subsequent DNA replication. By contrast, in strains in which RME1 is deleted or in strains that harbor the poorly expressed RME1-SK1A allele, m 6 A is dispensable for IME1 expression and subsequent DNA replication (Figs. 2e and 3a ). This observation positions IME4 as an upstream inhibitor of RME1 repression of IME1 (Fig. 3e ). This upstream placement explains previous observations that IME4 is required for IME1 induction in some strains but not in the SK1 strain [6] , [10] . This model in which IME4 functions upstream of RME1 for meiotic initiation is supported by epistasis analysis of DNA replication in the single and double IME4 and RME1 deletion strains. If IME4 and RME1 are in the same pathway, only one of the eight possible models is consistent with experimental data: IME4 represses RME1 , which represses DNA replication (Fig. 3a and Supplementary Table 3 ). Although ime4-Δ / ime4-Δ cells cannot replicate their DNA in the RME1-S288C background at any detectable level, ime4-cat / ime4-cat cells show only a ~75% reduction in DNA replication. Perhaps the effect of Ime4p on its target mRNAs is partially mediated through its interaction with the methylated transcript, in which case, m 6 A might function to stabilize this protein–RNA interaction. In this scenario, Ime4p-cat might still be able to bind its target mRNA with reduced affinity in the absence of its m 6 A catalytic activity, which would explain its intermediate phenotype compared to ime4-Δ . Our results show that the RME1 3′ UTR harbors a functional m 6 A site at +129A (Fig. 4d, e ): the rme1-10 mRNA that lacks the m 6 A site has significantly increased mRNA levels compared to wild-type RME1 mRNA (Fig. 5b ). As a result, IME4 / IME4 rme1-10 / rme1-10 cells have reduced DNA replication compared to IME4 / IME4 rme1-S288C / rme1-S288C cells. The single-nucleotide substitution in the RME1 3′ UTR accounts for ~1/3 to ~1/2 of the defect in ime4-cat / ime4-cat cells, validating the relevance of this m 6 A site to the meiotic program (Supplementary Fig. 5c and Fig. 5d ). The increase of RME1 mRNA levels in IME4 / IME4 rme1-10 / rme1-10 cells suggests a destabilizing effect for m 6 A on RME1 transcripts. This is consistent with a role for m 6 A in mRNA destabilization in mammals mediated by the reader protein YTHDF2 [29] , which has a homolog in yeast MRB1 [23] . Previous studies have used anti-m 6 A IP or anti-m 6 A crosslink IP followed by RNA-seq (m 6 A-seq and miCLIP, respectively) to map thousands of m 6 A sites in the transcriptomes of various cell types in numerous eukaryotes in which m 6 A plays developmental roles [13] , [15] , [21] , [22] , [23] , [24] . Despite this wealth of m 6 A data and the global effects of perturbing m 6 A deposition and recognition, little is known about the physiological relevance of individual m 6 A sites. However, at least three specific regulatory sites have been validated by mutational analysis: (1) An intronic m 6 A causes intron retention and rapid degradation of the SAM synthase mRNA when SAM levels are high; [25] , [50] (2) in the 5′ UTR of mammalian ATF4 mRNA, m 6 A directs upstream-open reading frame (ORF)-mediated alternative translation during amino acid starvation; [52] (3) in the 5′ UTR of mammalian HSP70 mRNA, m 6 A enables cap-independent translation during heat shock [51] . 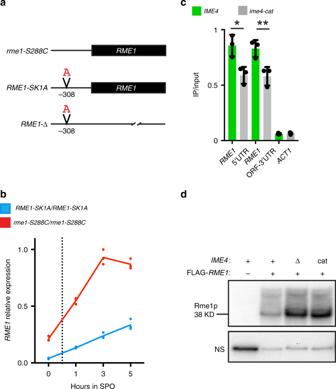Thus yeast RME1 provides the founding example of a consequential modification site within an mRNA 3′ UTR. Fig. 1 RME1alleles in this study.IME4downregulates Rme1p through its m6A activity.aThe threeRME1alleles are in the SK288C strain background.RME1-SK1Ahas a single A insertion 308 nucleotide upstream of the open reading frame (ORF) relative torme1-S288C.bQuantitative reverse transcription PCR (RT-qPCR) quantification ofRME1-SK1Aandrme1-S288Cexpression during meiosis. Means and individual values from three biological replicates. Source data are provided in a Source Data file.cm6A immunoprecipitation (IP) followed by RT-qPCR usingRME15′ untranslated region (UTR) primers or primers that span the end of the ORF and the 3′ UTR on mRNA isolated fromIME4andime4-cathomozygous cells, both inrme1-S288Chomozygous cells. Transcript levels were first normalized toPGK1as an internal control, and then the fold enrichment of IP/input was calculated. The residual enrichment ofRME1transcripts inime4-cat/ime4-catcells relative toIME4/IME4cells probably results from non-specific binding to the anti-m6A antibody13,23.ACT1serves as a non-methylated control. Means, individual values, and s.d. from three biological replicates. *p= 0.022, **p= 0.019, two-tailedttest. Source data are provided in a Source Data file.dWestern blot using anti-FLAG antibody showing Rme1p expression from therme1-S288Callele in strains homozygous for the indicated allelic backgrounds incubated in SPO media for 5 h. A non-specific (NS) band present in all lanes serves as a loading control. Source data are provided in a Source Data file Strains and sporulation Strain genotypes are shown in (Supplementary Table 1 ). Unless otherwise noted, all strains were constructed in the SK288C background [54] , [55] . To induce meiosis and sporulation, cells were grown in YPD (1% yeast extract, 2% peptone) supplemented with 4% glucose for 25 h at 30 °C with shaking and diluted to OD600 = 0.2 in BYTA media [66] (1% yeast extract, 2% tryptone, 1% potassium acetate, 50 mM potassium phthalate) and grown for an additional 16.5 h at 30 °C with shaking. Next, cells were washed once with water, re-suspended in SPO media (0.3% potassium acetate) to OD600 = 2, and incubated at 30 °C with shaking. RME1 phylogenetic analysis Sequence of the RME1 ORF and 500 nt upstream region in different strains of S. cerevisiae were obtained from aligned, assembled genomes from the Sanger Institute’s Saccharomyces Genome Resequencing project ( https://www.sanger.ac.uk/research/projects/genomeinformatics/sgrp.html ) using the alicat.pl tool, and the Sigma 1278b genome [67] . A maximum likelihood phylogenetic tree was generated with dnaml [68] and visualized with ClustalX [69] . Quantitative reverse transcription PCR RNA was extracted as follows: Frozen cells (~24 OD600) were disrupted by vortexing in 600 μl AE buffer (50 mM sodium acetate, 10 mM EDTA, 1% SDS) and 600 μl acid phenol (Fisher Scientific) in the presence of ~100 μl acid-washed glass beads (Sigma) at 4 °C for 5 min. RNA was extracted by incubation in phenol at 65 °C for 10 min. Next, cells were vortexed again as before, incubated at 65 °C for 10 min, vortexed, and spun down at 18,400 × g for 10 min at 4 °C. The aqueous top phase was transferred to a new tube and extracted again in phenol. After another spin down and transfer to a new tube, RNA was extracted in 400 μl chloroform followed by ethanol precipitation. 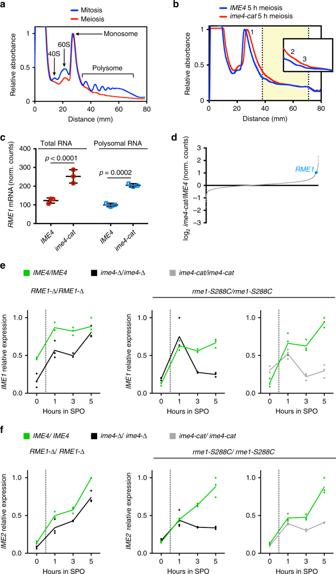cDNA was made with SuperScript III (Life Technologies) using random hexamers or gene-specific primers from 1 μg of total RNA. Fig. 2 IME4m6A activity reducesRME1mRNA levels to enable meiotic initiation.aPolysome profiles (absorbance at 254 nm vs. distance from the top of the tube) of mitotic cells during logarithmic growth and 2 h into meiosis. The locations of the 40S, 60S, monosome, and polysome peaks are indicated. Source data are provided in a Source Data file.bPolysome profiles of meioticIME4/IME4andime4-cat/ime4-catcells, both inrme1-S288C/rme-S288C. The inset is a magnification of the polysome area with the number of ribosomes in each peak. The highlighted area marks the pooled fractions used for RNA-seq of polysome-associated mRNA. Source data are provided in a Source Data file.cRNA-seq quantifications ofRME1transcript from input mRNA prior to gradient fractionation (total mRNA) and pooled polysome fractions (polysomal RNA) fromIME4/IME4andime4-cat/ime4-catmeiotic cells. Individual values, means, and s.d. from three biological replicates. Two-way analysis of variancepvalues are indicated. Source data are provided in a Source Data file.dRank order plot of mRNA levels in total RNA fromime4-cat/ime4-catandIME4/IME4meiotic cells. Means from three biological replicates. Source data are provided in a Source Data file.eLeft: Quantitative reverse transcription PCR (RT-qPCR) quantification ofIME1expression inRME1-Δ/RME1-Δduring meiosis inIME4/IME4andime4-Δ/ime4-Δcells. Middle: RT-qPCR quantification ofIME1expression inrme1-S288C/rme1-S288Cduring meiosis inIME4/IME4andime4-Δ/ime4-Δcells. Right: RT-qPCR quantification ofIME1expression inrme1-S288C/rme1-S288Cduring meiosis inIME4/IME4andime4-cat/ime4-catcells. Means and individual values from three biological replicates. Source data are provided in a Source Data file.fAs ineabove but with measurements ofIME2expression. Means and individual values from three biological replicates. Source data are provided in a Source Data file RT-pPCR was performed using SYBR green PCR master mix (Life Technologies) with primers listed in Supplementary Table 2 on Applied Biosystem 7500 or QuantStudio 5 instruments. Western blotting Ten OD600 of 2 OD/ml meiotic cells or cells grown to ~1 OD600/ml in YPD were collected by centrifugation, re-suspended in 1 ml water, spun down briefly, re-suspended in 5% w/v trichloroacetic acid, and incubated on ice for at least 10 min. Cells were then spun down at 18,400 × g for 2 min, and the supernatant was aspirated. The pellet was then washed in 500 μl non-pH-ed Tris to adjust the pH. After another centrifugation of cells and aspiration of the supernatant, the pellet was re-suspended in 140 μl of water. Next, 20 μl of 1 M DTT and 40 μl of 5× SDS loading buffer were added. Samples were then incubated for 5 min in a boiling water bath, put on ice, and vortexed just before gel electrophoresis using BioRad Criterion 10% Tris-HCl precast gels at 100 V for ~5–10 min and then at 120 V for ~90 min in Tris glycine SDS buffer. The gel was washed twice in water to remove SDS and equilibrated in transfer buffer (Tris glycine buffer with 15% methanol). Proteins were then transferred onto PVDF membranes (0.45-μM pore, Millipore) pre-incubated in methanol overnight at 15 V at 4 °C. Next, membranes were blocked in 5% milk in TBST (TBS buffer with 0.1% Tween 20) for 1 h at room temperature with shaking. Next, membranes were blotted with the following antibodies at the following dilutions in 5% milk TBST for 1 h at room temperature with shaking: M2 anti-FLAG-HRP (1:25,000, Sigma A8592-2MG), anti-Pgk1-HRP (1:500,000, Abcam 22C5D8), 10F3 anti-HA-HRP (1:10,000, Roche 12 013 819 001), and P4D1 anti-Ub-HRP (1:10,000, Enzo BML-PW0935-0025). Membranes were then briefly washed twice in TBST, followed by 5 more washes for 5 min each with shaking. Next, membranes were developed with supersignal West femto (Life Sciences) for 5 min before imaging with BioRad ChemiDoc XRS+ imaging system. For quantifications, a dilution series from each sample was first run to test signal linear range for each antibody. Proteins levels were then normalized to Pgk1p loading control using the Image J software. Uncropped and unprocessed blot images are in the Source Data file. Protein IP Cells from meiotic cultures incubated for 5 h in SPO were harvested by vacuum filtration and flash frozen in liquid nitrogen. Pellets were resuspended in 1 ml IP lysis buffer (50 mM HEPES pH 8.0, 150 mM NaCl, 1% Triton X-100, 0.1% deoxycholate, 5 mM EDTA, 1× cOmplete Mini EDTA-free protease inhibitor) and lysed by vortexing twice for 5 min with 200 μl acid-washed glass beads (Sigma) at 4 °C. Lysates were then cleared by centrifugation in a microcentrifuge at 21,100 × g for 10 min at 4 °C. Supernatants were transferred to new tubes and 40 μl were kept aside as input. In all, 25 μl per sample of M2 anti-FLAG magnetic beads (Sigma M8823) were washed twice in 200 μl IP lysis buffer and then added to each protein lysate sample followed by an overnight incubation on a rotating rack at 4 °C. The next morning, IP samples were washed 3 times in 900 μl ice-cold IP lysis buffer with vortexing and 5 min incubation on ice after each wash. Next, FLAG-Rme1p was eluted using 100 μg/ml FLAG peptide (Sigma) in lysis buffer. Three 100-μl elutions were done per sample and pooled. Eluted proteins were then precipitated by addition of 4 volumes of acetone pre-chilled overnight to −20 °C. Samples were incubated at −20 °C for 1 h and centrifuged at 15,000 × g for 10 min at 4 °C. Pellets were then washed in 1 ml chilled acetone and incubated at −20 °C for 1 h followed by another centrifugation as before. Next, protein pellets were dried in a biosafety hood, taking care not to over dry the pellets, and resuspended in 40 μl of purified water. Six microliters of 1 M DTT were added and samples were vortexed, then 11.5 5× sample buffer were added following by another vortex and boiling of samples prior to SDS-polyacrylamide gel electrophoresis and western blotting as described above. mRNA purification for m 6 A IP Total RNA was extracted from cells harvested by vacuum filtration and flash frozen in liquid nitrogen using hot acid phenol as described above. mRNA was purified by 2 rounds of polyA selection as follows: 50 μl of SeraMag Oligo dT magnetic beads (GE Healthcare) were used per 100 μg total RNA. RNA was diluted to 1 μg/μl using RNase-free water (Life Technologies). Beads were washed twice in 2× RNA-binding buffer (NEB #E7492AA) and re-suspended in 100 μl 2× RNA-binding buffer. 100 μl total RNA were then added and samples were vortexed gently. Samples were then incubated at 65 °C for 5 min followed by 5 min at 4 °C. After gentle vortexing, samples were placed on a rotating rack for 15 min at 25 °C. Next, beads were placed on a magnetic rack and the supernatant was removed. Beads were washed 3 times in 200 μl Wash buffer (NEB #E7493AA). Next, the supernatant was discarded and beads were resuspended 50 μl Tris buffer (NEB #E7496A). Samples were incubated at 80 °C for 2 min, then at 25 °C for 5 min. Next, 50 μl of 2× RNA-binding buffer were added and the samples were gently vortexed and placed on the rotating rack again for 15 min. Next, samples were placed on the magnetic rack and the supernatant was removed. Beads were washed twice in 200 μl Wash buffer. The Wash buffer was then removed with the magnetic rack. To ensure complete removal of the Wash buffer, samples were then centrifuged briefly, placed back on the magnetic rack, and residual buffer was removed. mRNA was then eluted by addition of 10 μl Tris buffer, mixing by pipetting, and incubating at 80 °C for 2 min, then immediately placing the tubes on the magnetic rack. mRNA was transferred to a new tube and 1 μl was used for size distribution evaluation with Agilent Bioanalyzer to ensure that the mRNA is intact. m 6 A IP for m 6 A-Seq m 6 A IP followed the procedure described in refs, [21] , [23] , [70] for three wild-type and three ime4-cat samples with some modifications as follows: mRNA purified as described above from meiotic cells incubated for 5 h in SPO was fragmented using RNA Fragmentation Reagents (Life Technologies) by incubation at 70 °C for 2 min in a total volume of 10 μl. This resulted in fragments mostly around 70–120 nucleotides long as assessed using an Agilent Bioanalyzer. The volume was raised to 100 μl with RNase-free water and ethanol precipitated with 2 μl Glycogen Blue (Life Technologies). Fragmented mRNA was re-suspended following ethanol precipitation in 13.5 μl RNase-free water. Then 0.5 μl Murine RNase inhibitor (NEB #M0314) was added, followed by 2 μl of 10× T4 polynucleotide kinase buffer (PKN, NEB #B0201), 1 μl T4 PKN enzyme (NEB #M0201), and 1 μl TURBO DNAse (Life Technologies). The total volume was 18 μl. Samples were then incubated at 37 °C for 30 min, and then 2 μl of 10 mM ATP were added and incubation resumed at 37 °C for another 30 min. This resulted in RNA fragments with a 5′-phosphate and a 3′-OH for subsequent library construction. 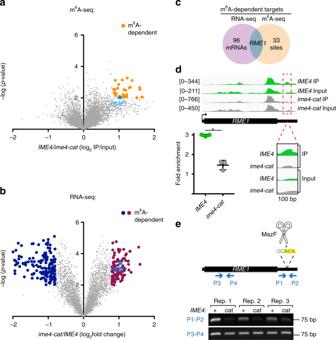Fig. 4 RME1mRNA harbors an m6A site at its 3′ untranslated region (UTR).am6A-seq data from meioticIME4homozygotes andime4-cathomozygotes. Data from three biological replicates are presented as immunoprecipitation (IP) to input ratio inIME4, divided by the same ratio inime4-cat. m6A sites enriched >1.75-fold inIME4relative toime4-catcells that have apvalue of <0.01 in a two-tailedttest are highlighted in orange.bRNA-seq data from meioticIME4homozygotes andime4-cathomozygotes cells. Data from three biological replicates are presented as normalized counts inime4-cat, divided by normalized counts inIME4. mRNAs increased >1.75-fold inime4-cat/ime4-catrelative toIME4/IME4cells (pvalue <0.01, two-tailedttest) are highlighted in purple. mRNAs decreased >1.75-fold inime4-cat/ime4-catrelative toIME4/IME4cells (pvalue < 0.01, two-tailedttest) are highlighted in blue.cVenn diagram showing the overlap between the m6A-seq data and the RNA-seq data.dRME1transcript with its 5′ and 3′ UTRs. IGV genome browser views of reads enriched following IP with anti-m6A antibodies inIME4/IME4andime4-cat/ime4-catcells are shown for the entire transcript (top, autoscale read counts on the left of each track), and in a 100-bp window of the 3′ UTR (bottom, reads in this window were normalized to input controls). Fold enrichment of IP/input for reads in the window are shown on the left with means and s.d. from three biological replicates. *p= 0.0006, two-tailedttest. Source data are provided in a Source Data file.ePCR amplification of cDNA prepared from MazF-digested meiotic mRNA fromIME4/IME4andime4-cat/ime4-catcells. Three biological replicates. P1 and P2 primer locations relative to the probed methylation site are indicated. The MazF ACA site within the methylation site is highlighted in yellow, and the probed nucleotide is marked with an asterisk. Primers P3 and P4, which do not flank an ACA site, were used as control. Source data are provided in a Source Data file 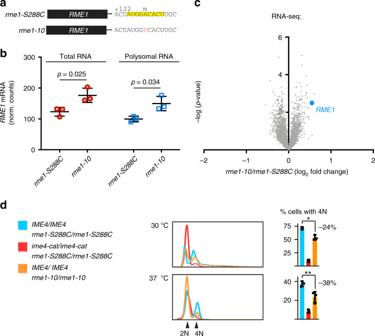Fig. 5 RME1methylation mutants are defective in meiotic DNA replication.arme1-S288Candrme1-10have the same promoter and coding sequence, but they differ in their 3′ untranslated region:rme1-10has a single A to T substitution of the +129 methylated A (marked with an m over it) in the methylation consensus motif (yellow).bRNA-seq quantifications ofRME1mRNA.RME1mRNA from input RNA prior to gradient fractionation (total mRNA) and polysome-associated RNA (polysomal RNA) fromIME4/IME4 rme1-S288C/rme1-S288CandIME4/IME4 rme1-10/rme1-10cells incubated in SPO media for 5 h. Individual values, means, and s.d. from three biological replicates. Two-way analysis of variancepvalues are indicated. Because this experiment was performed together with the one shown in Fig.2c, the results forRME1mRNA in theIME4background in Fig.2care re-plotted in this panel for therme1-S288Cbackground. Source data are provided in a Source Data file.cRNA-seq data fromrme1-S288Chomozygotes andrme1-10homozygotes incubated for 5 h in SPO media. Data from three biological replicates are presented as normalized counts inrme1-10, divided by normalized counts inrme1-S288C.dFlow cytometric analysis of DNA content over a meiotic time course inIME4/IME4 rme1-10/rme1-10compared toIME4/IME4 rme1-S288C/rme1-S288Candime4-cat/ime4-cat rme1-S288C/rme1-S288C. Cells were incubated for 24 h at 30 °C or 37 °C, as indicated. Means, individual values, and s.d. from three biological replicates. *p= 0.011, **p= 0.034, two-tailedttest. Source data are provided in a Source Data file The volume was then raised to 100 μl with RNase-free water and RNA was ethanol precipitated with 2 μl Glycogen Blue. Following ethanol precipitation, fragmented, end-repaired mRNAs were re-suspended in 100 μl IPP buffer (150 mM NaCl, 0.1% IGEPAL CA-630 [Sigma], 10 mM Tris-HCl, pH 7.5). Ten microliters were set aside as input. Twenty-five microliters of Protein G magnetic beads (NEB) per sample were washed twice in IPP buffer and then resuspended in IPP buffer. Two microliters of anti-m 6 A antibody (Synaptic Systems #202 003) per sample were added to the beads and incubated on a rotating rack at room temperature for 30 min. Next, beads were washed twice in IPP buffer, re-suspended in 25 μl IPP buffer per sample, and 2 μl of RNase OUT (Life Technologies) per sample were added and the beads were kept on ice. Ninety microliters of fragmented mRNA were incubated at 70 °C for 5 min, then added to the beads and incubated at 4 °C for 2 h on a rotating rack. Next, beads were washed three times in IPP buffer, transferred to a new tube, and washed two more times. The beads were then centrifuged briefly and returned to the magnetic rack to remove residual IPP buffer. Antibody-bound RNA was then eluted using 30 μl of RLT buffer (Qiagen). Next, input and IP samples volumes were made up to 100 μl with RNase-free water, and RNA was ethanol precipitated with 2 μl Glycogen Blue. Input and IP samples were re-suspended in 7 μl of RNase-free water. One microliter was used for determining RNA concentration with Agilent Bioanalyzer and the rest were used for library construction using NEBNext Multiplex Small RNA Library Prep Set of Illumina with primer set 2 (NEB #E7580S), according to the kit’s instructions. Adapters were diluted 1:3 and libraries were amplified with 15 PCR cycles. Libraries were run on an Agilent Bioanalyzer HS DNA chip, and using this data, the libraries were subsequently pooled so that the amounts of material between 160 and 270 bp were equal (ng). The final pooled library was size-selected on a PippinHT using a protocol set to elute from 140 to 280 bp, ensuring that fragments within the target of 160–270 bp were captured. Following pooling of barcoded libraries, products were size selected to 140–270 bp using a Pippin prep and sequenced on an Illumina HiSeq generating 75 × 75 paired end reads. UTR extensions All reads were quality controlled and adaptors removed using FASTX Toolkit (v 0.0.14) and cutadapt (v1.16). Since the Ensembl R64-1-1-80 (sacCer3) transcriptome annotations do not include UTRs, we computationally extended canonical gene 5′ and 3′ UTRs using RNA-Seq data from S. cerevisiae SK288C 5 h meiotic cells. Using bowtie2 (v2.3.4.1), we mapped reads to the Ensembl R64-1-1-80 (sacCer3) genome in a strand-specific fashion and calculated per-base coverage for each annotated gene using the bedtools commands “bamtobed” and “genomeCoverageBed” [71] . The strand-specific per-base coverage was used to extend each UTR one base at a time until the coverage fell below 1/3 of the ORF’s median coverage, intersected an adjacent ORF, or reached 500 nt. UTR length was defined as the median length across all six input samples (three wild-type and three ime4-cat replicates). Read alignment Reads were subsequently mapped against the Ensembl R64-1-1-80 (sacCer3) genome using Tophat2 (v2.1.1) [72] with a custom GTF file of the transcriptome that including UTR extensions (as defined above). In addition, we used the options “–max-multihits 1–prefilter-multihits.” To connect each read pair, the Tophat2 output bam file was converted into a bedpe file with bedtools (v2.27) and this file was subsequently used to calculate per base coverages for each gene by using bedtools “genomeCoverageBed” [73] . Detection of m 6 A sites Detection of m 6 A sites followed the procedure outlined in ref. [23] . Briefly, putative m 6 A sites were identified using the following method: (1) Examination of the IP samples to identify m 6 A peaks within annotated genes including UTR extensions that were enriched compared to overall gene levels. (2) Comparison of IP to input enrichments (for wild-type and ime4-cat samples) to identify IP-specific peaks not present in inputs. (3) Comparison of wild-type and ime4-cat samples to identify WT-specific peaks not present in ime4-cat . 1. Peak detection: Genes with median expression >0 in all six IP samples were analyzed for potential m 6 A peaks. To identify peaks in the IP samples, each gene was scanned using sliding windows of 100 bases with a 50-base overlap. Each window was scored by calculating the mean coverage across the window divided by the median coverage of the gene. Windows having an enrichment score of >3 and a mean read depth of >10 were identified as peaks. 2. Identification of IP-specific peaks: The peak detection step was repeated for each input sample. Peaks present in IP and not in input were retained for all subsequent analyses. 3. Identification of wild-type-specific peaks: All peaks passing steps 1 and 2 in at least one sample were retained, and adjacent peaks were merged. For each merged peak, we recalculated the enrichment score as defined in step 1. m 6 A-dependent peaks were defined as those with a wild-type enrichment score divided by the ime4-cat enrichment score of at least 1.75, with the remaining peaks described as m 6 A independent. The summit of each peak was defined as the position with the highest coverage. Motif mapping and distance to the nearest motif We calculated the distance from each of the 118 peak summits enriched in at least 2-fold in wild type compared to ime4-cat to the nearest RGAC motif on the same strand. As a control, we used 118 randomly selected summits from the m 6 A-independent peaks. As described in ref. [23] , we identified 58 m 6 A-dependent summits within 5 nt of the nearest RGAC motif, extracted 24 nt centered on this motif, and used those as inputs for MEME (v5.0.0) [74] to determine the consensus m 6 A motif. Metagene m 6 A-gene distribution The position of each of the 118 m 6 A-dependent peak summits was expressed as a fraction of the corresponding gene’s transcript length. As a control, we performed the same analysis on the lowest scoring 118 m 6 A-independent peak summits. Gene ontology GO categories analysis was carried using YeastMine (yeastmine.yeastgenome.org). m 6 A IP for RT-qPCR Total RNA from meiotic cells incubated for 5 h in SPO was prepared as described above. One hundred micrograms of total RNA were spiked with 10 pg of in vitro transcribed Luciferase polyadenylated mRNA (Promega) for normalization, and mRNA was purified as described above and assayed using an Agilent Bioanalyzer. IP was done in the same way as for m 6 A-seq, except that intact rather than fragmented mRNA was used. cDNA from input and IP samples was generated with SuperScript III (Life Technonolgies) using 200 ng of mRNA. RT-pPCR was performed using SYBR green PCR master mix (Life Technologies) with primers listed in Supplementary Table 2 on an Applied Biosystem QuantStudio 5 instrument. Polysome profiling All cultures were rapidly harvested by vacuum filtration and flash frozen in liquid nitrogen. Frozen pellets were mechanically lysed using a Sample Prep 6870 Freezer/Mill (Spex SamplePrep; 10 cycles of 2 min on, 2 min off at setting 10). Lysate powder was aliquoted and stored at −80 °C. Crude lysates were prepared by re-suspending an aliquot of thawed lysate powder (approximately 800 μl of loosely packed powder, kept on ice for 3 min before re-suspension) in 1 ml of lysis buffer (10 mM Tris-HCl [pH 7.4], 5 mM MgCl 2 , 100 mM KCl, 1% Triton X-100, 1% Sodium Deoxycholate, 2 mM DTT, 0.4 mM cycloheximide, 20 U/ml SUPERase•In [Ambion], cOmplete EDTA-free Protease Inhibitor Cocktail [Roche]). The lysates were placed on a rotator mixer at 4 °C for 5 min to allow for re-suspension. Following brief vortexing, lysates were centrifuged at 1300 × g for 10 min, and 800 μl of the supernatant was loaded onto a 12.5 ml linear 10–50% (w/v) sucrose gradient (20 mM HEPES-KOH [pH 7.4], 5 mM MgCl 2 , 100 mM KCl, 2 mM DTT, 0.4 mM cycloheximide, 20 U/ml SUPERase•In). Gradients were centrifuged in a pre-chilled SW-41 Ti rotor at 222,000 × g r max (acceleration mark “1,” deceleration mark “7”) for 2 h at 4 °C. Gradients were fractionated using a Piston Gradient Fractionator (Biocomp) in 1 ml fractions. A 254 was monitored using an Econo UV Monitor (Biorad) and Gradient Profiler software (Biocomp, v2.07). Polysome fractions from each sample were pooled. SDS (2%) with 40 μg/ml Proteinase K in RNase-free water was added 1:1 to pooled polysome or re-suspended input lysate in 15-ml conical tubes, followed by incubation for 30 min at 42 °C in an Eppendorf Thermomixer with shaking at 550 rpm. Then 2 ml of acid phenol were added and the samples were vortexed and incubated at 42 °C for another 5 min. Samples were then transferred to new tubes and spun down at 9400 × g for 10 min. The aqueous phases were transferred to new tubes and extracted with 2 ml chloroform followed by another vortex and centrifugation as before. The aqueous phases were moved to new tubes and RNA was precipitated by adding 200 μl sodium acetate, vortex, 4 μl Glycogen Blue (Life Technologies), vortex, and 2 ml isopropanol followed by overnight incubation at −20 °C. The next day, samples were centrifuged and RNA was re-suspended in 1 ml 70% ethanol in RNase-free water and moved to 1.5 ml microcentrifuge tubes, followed by 30 min centrifugation at 18,400 × g at 4 °C. RNA samples were re-suspended in RNase-free water. mRNA from total RNA prior to gradient fractionation and from pooled polysomal fractions was purified as described above and used for library construction with the NEBNext Ultra RNA Library Prep Kit for Illumina (#E7530S), according to the manufacturer’s instructions. MazF mRNA restriction followed by PCR assay Two hundred nanograms of polyA-selected mRNA from 5 h meiotic cells were denatured at 70 °C for 2 min and placed on ice. Next, 4 μl MazF buffer and 0.5 μl RNase inhibitor (NEB, M0314L) were added, and the volume was made up to 19 μl with RNase-free water. Next, 1 μl (20 U) of MazF (TaKaRa 2415A) were added and the samples were incubated at 37 °C for 2 h before ethanol precipitation with glycogen blue as described above. Next, RNA was resuspended in 8 μl RNAse-free water and cDNA was synthesized using SuperScript III with random hexamers (Life Technologies 18080–051) according to the manufacturer’s instructions. Two microliters of the resulting cDNA were used in subsequent PCR reactions using EmeraldAmp GT PCR master mix (TaKaRa RR310), and the products were run on a 2% agarose TBE gel stained with SYBER safe (Life Technologies S33102). Flow cytometric measurements of DNA replication Five hundred microliters of meiotic cells were fixed in 1.5 ml 100% EtOH for at least 1 h in room temperature or overnight at 4 °C. Cells were then spun down briefly and re-suspended in 500 μl of 50 mM sodium citrate containing 40 μg/ml RNase A (Sigma), vortexed, and incubated at 50 °C for 1 h. Next, 10 μl of 20 μg/μl Proteinase K (Life Technologies) were added to each sample for another 1 h incubation at 50 °C followed by vortexing. Five hundred microliters of SYTOX green (Life Technologies) diluted 1:250 in 50 mM sodium citrate were then added to each sample. After vortexing, cells were transferred to 5 ml FACS tubes and analyzed using a BD CantoII instrument and BD FACS Diva software. Single cells were gated based on forward and side scattering, FITC-A, and FITC-W. Ten thousand events were counted per sample. Data were analyzed using the FlowJo 10 software. Meiotic division assay Two hundred microliters of meiotic cells incubated for 24 h in SPO media were fixed in 500 μl 100% ethanol for at least 1 h at room temperature. Cells were centrifuged briefly and resuspended in 100 μl of 1 μg/ml DAPI in water and imaged using Nikon Eclipse Ti fluorescence microscope at ×100 magnification. Cells were counted and the percentage of cells with more than one nucleus was calculated. Sporulation assay Two hundred microliters of meiotic cells incubated for 48 h in SPO media were fixed in 500 μl 100% ethanol for at least 1 h at room temperature. Cells were centrifuged briefly and resuspended in 100 μl water and imaged using Nikon Eclipse Ti fluorescence microscope at ×100 magnification. Cells were counted and the percentage of asci was calculated. Statistics and reproducibility All statistical data were calculated using GraphPad Prism 7. Comparisons of data in Figs. 2c and 4f were performed using two-way analysis of variance. Fisher’s Exact Test was used for Supplementary Fig. 4d . For all other comparisons, two-tailed t tests were used. All experiments were repeated three times or performed in triplicates unless otherwise indicated. Reporting summary Further information on research design is available in the Nature Research Reporting Summary linked to this article.